Crystal Structures ofWolbachiaCidA and CidB Reveal Determinants of Bacteria-induced Cytoplasmic Incompatibility and Rescue Cytoplasmic incompatibility (CI) results when Wolbachia bacteria-infected male insects mate with uninfected females, leading to embryonic lethality. “Rescue” of viability occurs if the female harbors the same Wolbachia strain. CI is caused by linked pairs of Wolbachia genes called CI factors (CifA and CifB). The co-evolution of CifA-CifB pairs may account in part for the incompatibility patterns documented in insects infected with different Wolbachia strains, but the molecular mechanisms remain elusive. Here, we use X-ray crystallography and AlphaFold to analyze the CI factors from Wolbachia strain w Mel called CidA w Mel and CidB w Mel . Substituting CidA w Mel interface residues with those from CidA w Pip (from strain w Pip) enables the mutant protein to bind CidB w Pip and rescue CidB w Pip -induced yeast growth defects, supporting the importance of CifA-CifB interaction in CI rescue. Sequence divergence in CidA w Pip and CidB w Pip proteins affects their pairwise interactions, which may help explain the complex incompatibility patterns of mosquitoes infected with different w Pip strains. Wolbachia pipientis is an intracellular bacterium infecting ~40% of all terrestrial arthropod species and certain filarial nematodes [1] , [2] , [3] . They are primarily inherited maternally [4] . Their remarkable success in spreading in arthropod populations is in part driven by the ability of Wolbachia to increase the number of infected females [5] , often by acting as reproductive parasites that distort host sex ratios or reproductive outcomes [6] . The most common type of reproductive parasitism is cytoplasmic incompatibility (CI) [6] , which is a type of post-zygotic male sterility characterized by improper paternal chromatin condensation and separation in the first mitosis cycle [7] , [8] , [9] . CI causes Wolbachia- infected male insects to be sterile in matings with uninfected females but not similarly infected females (called ‘rescue’), providing a selective advantage for infected females and thus driving Wolbachia into the host population [6] , [10] . Insect species infected by two or more different Wolbachia strains can be bidirectional incompatible [11] , [12] , [13] , which causes reproductive isolation of populations infected with different strains [11] , [14] . Based on the outcomes of crosses between Wolbachia- infected insects, it has been proposed that CI is governed by a modification-rescue system [15] , [16] . Specifically, a modification activity from Wolbachia is postulated to modify sperm during spermatogenesis, and a rescue activity in the infected egg reverses or neutralizes the original sperm modification following fertilization. The existence of both unidirectional and bidirectional incompatibilities in infected insect populations has led to agreement that Wolbachia may carry multiple modification and rescue factors [12] , [13] , but the molecular identity of these factors remained unknown for nearly half a century [17] , [18] , [19] , [20] . Recently, the key factors involved in CI induction and rescue were identified [21] , [22] , [23] , [24] . They are known as CI factors or Cifs, which are encoded by pairs of linked genes, cifA and cifB . Transgenic expression of both cifA and cifB genes, or cifB alone, in the germline of male Drosophila melanogaster or Anopheles gambiae , induces sterility that is highly similar to CI induced by Wolbachia [21] , [22] , [25] , [26] , [27] . This embryonic lethality can be rescued by crossing transgenic males with Wolbachia- infected females or those with a transgenic cifA gene expressed in the germline [22] , [23] , [24] . The cif genes have diverged into at least five distinct phylogenetic groups, which are named types I-V [22] , [28] , [29] , [30] . The degree of similarity and the presence/absence of cif gene homologs between Wolbachia strains correlates with known patterns of bidirectional incompatibility. For instance, Wolbachia strain w Ri is able to rescue w Mel-induced CI in same-species crosses, probably because these two strains share highly related type-I homologs of the cifA gene (99% amino acid identity); however, the reverse is not true: w Mel cannot rescue w Ri-induced CI, likely due to w Ri also encoding a type II gene pair that is much more divergent [12] , [13] , [24] . In general, the cif genes from bidirectionally incompatible Wolbachia pairs are highly divergent, with only 29–68% amino-acid identity [22] . Recent analysis of transgenic cif gene expression in D. melanogaster is largely consistent with this view [31] . The cifA and cifB genes are coevolving [22] , [30] , [32] . Protein-binding experiments and expression of cif genes in yeast have shown that CifA binds its cognate CifB specifically and rescues CifB-induced yeast growth defects [21] , [23] . Although the specific roles of cifA and cifB in CI induction and rescue are still not fully understood, the co-divergence of the cifA and cifB genes [22] , [32] , [33] has been proposed to be partially responsible for bidirectional incompatibility, possibly by modulating CifA-CifB binding [34] , [35] . Among the five types of cif genes, only type I and certain type V cifB genes encode a deubiquitylase (DUB) domain [21] . (Hereafter, we will use “Cif” for the entire set of CI factors and “Cid” for the deubiquitylase family and primarily focus on the type I Cid protein family.) The cidA and cidB genes from Wolbachia strains w Mel (hereafter cidA w Mel and cidB w Mel ) and w Pip (hereafter cidA w Pip and cidB w Pip ) are among the most well studied cif genes (Fig. 1a ). These Wolbachia strains are expected to be incompatible, as shown by crosses between trans-infected Aedes albopictus mosquitoes [36] . Unlike the w Mel strain, Wolbachia w Pip strains found in different populations of Culex pipiens are highly diversified. Many of them carry several polymorphic copies of the cidA w Pip and cidB w Pip genes, which may function as independent modification and rescue factors and associate with the diverse CI phenotypes in w Pip-infected C. pipiens [32] , [37] . Thus, the Cid proteins can be used as a model to study how the diversification of cidA w Pip and cidB w Pip affects protein-protein interactions and how it is related to CI induction and rescue. Fig. 1: Crystal structures of CidA w Mel and CidB w Mel DUB , and a model of CidB w Mel ND1-ND2 reveal the molecular basis for CI. a CidA w Mel and CidB w Mel , and CidA w Pip and CidB w Pip form alternative two-gene CI systems. Each domain is assigned a unique color. b CidA w Mel contains mostly α-helices. The C-terminal domain contains six HEAT repeats (HR1-HR6). Residues 111-154 and 158-165 are disordered. c CidB w Mel DUB consists of a five-stranded β sheet flanked by α helices on both sides. The active center residues are labeled and shown as balls and sticks. d A model for CidB w Mel ND1-ND2 was built with AlphaFold. e The crystal structure of the CidA w Pip(Tunis) -CidB w Pip(Tunis) ND1-ND2 complex. NTD: N-terminal domain; CTD C-terminal domain; ND nuclease domain; DUB deubiquitylase domain; AA amino acids; HR HEAT repeats. Full size image Here, we report crystal structures for CidA w Mel and the DUB domain of CidB w Mel and build a model of the CidA w Mel -CidB w Mel complex using AlphaFold-Multimer [38] , which is validated and confirmed by comparison to a crystal structure of a homologous CidA w Pip -CidB w Pip complex. Substituting the CidA w Mel residues at the CidB-binding interfaces with those of CidA w Pip enables it to bind CidB w Pip and rescues CidB w Pip -induced yeast growth defects, which suggests a role of cid gene co-evolution in modulating CidA-CidB binding specificity. Analysis using the crystal structures of the CidA w Pip -CidB w Pip complex further shows that sequence divergence in Wolbachia w Pip may result in complex binding patterns between Cid w Pip protein variants. These results provide a solid base for future investigations of CI mechanism and shed light on how co-evolution of CidA-CidB pairs modulates their interactions and bidirectional CI. 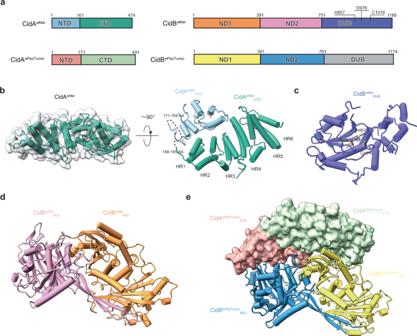Fig. 1: Crystal structures of CidAwMeland CidBwMelDUB, and a model of CidBwMelND1-ND2reveal the molecular basis for CI. aCidAwMeland CidBwMel, and CidAwPipand CidBwPipform alternative two-gene CI systems. Each domain is assigned a unique color.bCidAwMelcontains mostly α-helices. The C-terminal domain contains six HEAT repeats (HR1-HR6). Residues 111-154 and 158-165 are disordered.cCidBwMelDUBconsists of a five-stranded β sheet flanked by α helices on both sides. The active center residues are labeled and shown as balls and sticks.dA model for CidBwMelND1-ND2was built with AlphaFold.eThe crystal structure of the CidAwPip(Tunis)-CidBwPip(Tunis)ND1-ND2complex. NTD: N-terminal domain; CTD C-terminal domain; ND nuclease domain; DUB deubiquitylase domain; AA amino acids; HR HEAT repeats. Crystal structures of CidA w Mel and CidB w Mel DUB , and a model of CidB w Mel ND1-ND2 We determined the crystal structure of CidA w Mel to 2.75 Å resolution (Supplementary Table 1 ). CidA w Mel is made up largely of α-helices (Fig. 1b ). Residues 111-154 and 158-165 are disordered and cannot be modeled, which divide CidA w Mel into an N-terminal domain (NTD, residues 1 to 161) (see below for why we include these disordered residues as part of the N-terminal domain) and a C-terminal domain (CTD, residues 162 to 422) (Fig. 1b ). The C-terminal domain folds into a twisted set of six HEAT repeats, a structural motif that primarily mediates protein-protein interactions [39] (Fig. 1b ). CidB w Mel was expressed poorly in Escherichia coli , making direct structure determination difficult. We used a “divide-and-conquer” strategy to obtain structural information for each of its domains separately. CidB w Mel consists of a region, which is predicted to contain two PD-(D/E)XK (pseudo) nuclease domains (residue 1-751; hereafter CidB w Mel ND1-ND2 , ND: nuclease domain) and a C-terminal deubiquitylase (DUB) domain. An active DUB domain is required for inducing a CI-like phenotype in transgenic D. melanogaster for cid operons [21] . We determined the crystal structure of the CidB wMel DUB domain to 1.85 Å resolution (Supplementary Table 1 and Fig. 1c ). Similar to the structures of other proteases in the CE clan/Ulp1-like protease family [40] , [41] , the DUB core consists of a five-stranded β sheet flanked by α helices on both sides. His957, Asp976, and Cys1016 form the catalytic triad (Fig. 1c ). Three variable regions (VRs), a constant region (CR) and a C-terminal accessory domain may account for the S1 ubiquitin-binding interface [41] (Supplementary Fig. 1a-d ). A model for CidB w Mel ND1-ND2 (Fig. 1d ) was built with the AlphaFold [42] program. Although the predicted structural model has an average pLDDT score as high as 83.190, which confirms its quality (pLDDT > 70 indicates the backbone prediction is correct [43] ), we wanted to validate this model further. CidB w Mel ND1-ND2 shares sequence homology with other CifB molecules [34] . Of note, the ND1-ND2 region of CidB w Pip _I(b/2) (a CidB w Mel ortholog from the Wolbachia strain w Pip Tunis line [30] , hereafter CidB w Pip(Tunis) ND1-ND2 ) expressed well in E. coli and shares a sequence identity of 71% with CidB w Mel ND1-ND2 (Supplementary Fig. 2 ). We successfully determined a crystal structure of CidB w Pip(Tunis) ND1-ND2 in complex with CidA w Pip(Tunis) (specifically CidA w Pip _I(γ/2) [32] ) (Supplementary Table 1 , Figs. 1e and 2a ). The structure of CidB w Pip(Tunis) ND1-ND2 could be used for comparison with CidB w Mel ND1-ND2 modeled by AlphaFold [42] . Fig. 2: CidA and CidB interact through a large conserved tripartite interface. a The structure of the CidA w Pip(Tunis) -CidB w Pip(Tunis) ND1-ND2 complex. CidA w Pip(Tunis) binds CidB w Pip(Tunis) ND1-ND2 through three regions (Interface I, II, and III). b A structural model of CidA w Mel in complex with CidB w Mel ND1-ND2 was generated by AlphaFold-Multimer. The tripartite interface between CidA w Mel and CidB w Mel ND1-ND2 is shown in yellow, magenta and cyan for Interface I, II, and III, respectively. c – e Each interface of the CidA w Mel -CidB w Mel ND1-ND2 complex involves a pair of structural motifs. Representative residues directly involving in the interaction are labeled and shown as balls and sticks. f – h The structural motifs at Interface I, II and III of the CidA w Pip(Tunis) -CidB w Pip(Tunis) ND1-ND2 complex are shown, with residues directly involving in the interaction labeled. NTD N-terminal domain; CTD C-terminal domain; ND nuclease domain. Full size image The structure of CidB w Pip(Tunis) ND1-ND2 is very similar to the model for CidB w Mel ND1-ND2 (Supplementary Fig. 3a ). Moreover, the residues that are varied among CidB homologs are mainly located at the surfaces of the protein (Supplementary Fig. 4a ), which should not affect protein folding. Thus, the model for CidB w Mel ND1-ND2 is likely to be accurate. Since the cif genes from w Mel have been well characterized, we will mainly focus on the structures and functional analysis of the CidA w Mel -CidB w Mel ND1-ND2 pair in the following sections. The results from the CidA w Pip(Tunis) -CidB w Pip(Tunis) system will be mentioned when necessary. CidB w Mel ND1-ND2 consists of two NDs; ND1 comprises residues 1-391 and ND2 comprises residues 392-751 (Fig. 1d ). The ND1 and ND2 domains of CidB w Mel interact through an extensive interface burying a surface area of ~2200 Å 2 . This interface is highly similar to that of CidB w Pip(Tunis) (Supplementary Fig. 3b-c ) and the residues involving in ND1-ND2 interaction are highly conserved among CidB homologs (Supplementary Fig. 3d-f ). Interestingly, in addition to the (inactive) PD-(D/E)XK modules predicted by sequence homology analysis (residues 277-375 and 607-730) [21] , [28] , [29] , [30] , the structural model of CidB w Mel shows that each ND has an additional more divergent PD-(D/E)XK module (residues 30-137 and 431-523) (Supplementary Fig. 5 ). None of these modules present the key canonical catalytic residues E-D-E-K [23] (the putative corresponding residues are P33, K77, S92, S94 in module I, K279, Y311, N330, T332 in module II, F435, K475, I491, D493 in module III and K609, G663, V680, G682 in module IV based on structural analysis (Supplementary Fig. 5 )). These modules may play structural roles or support an alternative catalytic activity. CidA w Mel binds CidB w Mel through a large distinct interface We built a model for the CidA w Mel -CidB w Mel ND1-ND2 complex using AlphaFold-Multimer [38] (Fig. 2b ). The predicted end-to-end structure has a ranking score (TM-Score) as high as 0.8568 with a ptm score (intra-chain quality) of 0.86436 and an iptm score (interface score) of 0.85498. This indicates our prediction is highly reliable both for the protein themselves and the interface between them. The obtained end-to-end model was further optimized by Molecular Dynamics (MD) simulations. Two independent trajectories were performed and both achieved equilibrium within the first 100 ns and were then trapped in optima in the next 100 ns. The Root-Mean-Square Deviation (RMSD) for one of the simulation trajectories was recorded (Supplementary Fig. 6a ). Trajectory cluster analysis was performed and the most stable binding conformation was extracted from the largest cluster of the trajectory as the final binding complex of CidA w Mel -CidB w Mel ND1-ND2 . The complex also predicts many hydrogen bonds and salt bridges between CidA w Mel and CidB w Mel ND1-ND2 at the three interfaces (Fig. 2c–e ) and only 0.57% of the residues are Ramachandran outliers (Supplementary Fig. 6b ), which demonstrated the side chains of the predicted model have been reliably predicted. Therefore, we believe that the model of the CidB w Mel ND1-ND2 and its complex with CidA w Mel is reasonable. The interface between CidA w Mel and CidB w Mel ND1-ND2 can be divided into three regions (Fig. 2b ); each region mainly involves a pair of structural motifs. At the first region (Interface I), the helices consisting of the residues 93-158 of CidA w Mel interact with a loop in CidB w Mel ND1-ND2 (residues 448-462) through a network of hydrogen bonds and salt bridges (Fig. 2c ). Interestingly, the region of CidA w Mel which is disordered in the absence of CidB w Mel (residue 111-154 and 158-165) is modeled to form a helix bundle upon complex formation (Figs. 1b and 2c ), consistent with its role in mediating CidA w Mel -CidB w Mel ND1-ND2 interaction. These residues are part of the N-terminal domain. Interface II is formed by the helices at the N-terminus of CidA w Mel (residues 2-60) and helices from both NDs of CidB w Mel ND1-ND2 (residues 337-353 and 395-418) (Fig. 2d ). Interface III involves multiple HEAT repeats in CidA w Mel and a cross-cutting helix (residues 241-264) in CidB w Mel ND1-ND2 that is bolstered by two β strands and their connecting loop (residues 365-387) to stabilize the interaction (Fig. 2e ). Interestingly, although the model of CidA w Mel -CidB w Mel ND1-ND2 complex is very similar to the structure of CidA w Pip(Tunis) -CidB w Pip(Tunis) ND1-ND2 (Fig. 2a, b ), the residues involving in interaction at the three interfaces are very different between the two complexes (Fig. 2c–h ), which could help explain their cognate-specific binding. (The residues at the interface are well resolved in CidA w Pip(Tunis) -CidB w Pip(Tunis) ND1-ND2 with good electron density (Supplementary Fig. 7 )). Pulldown experiments and yeast growth assays were used to validate these structural models. As a model system, it has been demonstrated that expression of cidB genes in the yeast S accharomyces cerevisiae inhibits cell growth, but growth is at least partially restored if the cognate cidA gene is coexpressed, resembling CI induction and rescue in insects [21] , [23] . Substituting the CidA w Pip(Tunis) residues at its CidB-binding interface with the corresponding ones from CidA w Mel abolished its ability to bind CidB w Pip(Tunis) ND1-ND2 and neutralize the CidB w Pip(Tunis) -induced growth defect in yeast (Supplementary Fig. 8 ). Thus, the structure of the CidA w Pip(Tunis) -CidB w Pip(Tunis) ND1-ND2 complex accurately captures the CidA-CidB interaction mode and is biologically relevant. However, due to the poor expression of CidB w Mel ND1-ND2 in E. coli and the low toxicity of CidB w Mel in yeast, we could not directly validate the model of the complex by pulldown or yeast growth analysis. To test the reliability of this model, we rationally designed a set of mutations based on the model to demonstrate that the interaction mode is conserved between the w Pip and w Mel CidA-CidB pairs (see below). CidA-CidB binding specificity is determined by residues at their interfaces Until now, only CifA and CifB proteins expressed from the same operon have been shown to interact [21] , [23] , [35] . The specific interactions between CifA and CifB have been proposed to play a role in CI induction and/or rescue, depending on different CI models. We substituted multiple residues at the binding interface of CidA w Mel with the corresponding region of CidA w Pip(Tunis) (Fig. 3a–c ) and investigated if the chimeric construct (named CidA w Mel (ST)) could now bind CidB w Pip(Tunis) ND1-ND2 . Their interaction, while detectable, was weak, probably because the residues substituted are not the major binding determinants for interaction between CidA w Pip(Tunis) and CidB w Pip(Tunis) ND1-ND2 (Fig. 3d ). Interestingly, CidA w Mel (ST) could bind a closely related CidB w Pip ND1-ND2 from Wolbachia strain w Pip(Pel) (hereafter CidB w Pip(Pel) ND1-ND2 ) to an extent similar to the binding of the cognate CidA w Pip(Pel) (Fig. 3d , lane 2 vs. lane 4). By contrast, CidA w Mel had been shown previously to be unable to bind CidB w Pip(Pel) (Ref. 21 ). CidB w Pip(Pel) ND1-ND2 only differs from CidB w Pip(Tunis) ND1-ND2 by 30 residues (Supplementary Fig. 9 ). We used CidB w Pip(Pel) for further biochemical investigation. Fig. 3: Mutagenesis with binding and yeast growth assays reveal how residues at the three interfaces determine CidA binding specificity. a , b CidA w Mel (ST) is a chimera with the body of CidA w Mel (pink) and interfacial residues from CidA w Pip(Tunis) . The locations of the mutated residues are shown in orange on the CidA w Mel structure. c The substituted residues in CidA w Mel (ST) are divided into nine regions (R) and reversed back to those of CidA w Mel , individually, to create CidA w Mel (ST-1) through CidA w Mel (ST-9). d CidA w Mel (ST) does not bind wild-type CidB w Mel but binds CidB w Pip(Pel) to a similar extent as CidA w Pip(Pel) . Regions 4, 7, and 9 play important roles in binding. The experiment was repeated three times independently with similar results obtained. One representative is shown. e CidA w Mel (ST) is able to rescue yeast from CidB w Pip(Pel) -induced lethality. f CidA w Mel (ST-4), CidA w Mel (ST-7) and CidA w Mel (ST-9), which do not bind CidB w Pip(Pel) , also fail to suppress CidB w Pip(Pel) -induced yeast growth defects. g The crystal structure of the CidA w Mel (ST)-CidB w Pip(Pel) ND1-ND2 complex is similar to the model of the CidA w Mel -CidB w Mel ND1-ND2 complex. Representative residues directly involved in the CidA w Mel (ST) and CidB w Pip(Pel) ND1-ND2 interactions at Interface ( h ) I and ( i ) III are labeled. ST substituted; ND nuclease domain. Source data for panels ( d ) and ( e ) are provided as a Source Data file. Full size image Agreeing with the pulldown experiments, yeast growth defects induced by CidB w Pip(Pel) could be rescued by both CidA w Mel (ST) and CidA w Pip(Pel) , but not CidA w Mel (Fig. 3e ) even though the expression levels for CidA w Mel and CidA w Mel (ST) were similar (Supplementary Fig. 10 ). These data clearly show the importance of the interfacial residues (Fig. 3e ) in determining binding specificity. They also support the accuracy of our CidA w Mel -CidB w Mel ND1-ND2 model. To locate the critical regions that determine binding specificity, the substituted interfacial residues of CidA w Mel (ST) were divided into nine groups/regions based on their location in the primary sequence and three-dimensional structure. Each region was individually reverted back to the original sequence in CidA w Mel (Fig. 3b, c ), resulting in CidA w Mel (ST-1) to CidA w Mel (ST-9). (Regions 1, 2 are at Interface II. Regions 3, 4, 5, 6 are at Interface I. Regions 7, 8, 9 are at Interface III.) CidA w Mel (ST-4), CidA w Mel (ST-7) and CidA w Mel (ST-9) showed reduced binding affinity to CidB w Pip(Pel) ND1-ND2 (Fig. 3d ). They also failed to rescue CidB w Pip(Pel) -induced yeast growth defects (Fig. 3f ). (These CidA variants were expressed at similar levels. Interestingly, however, co-expression of CidA w Mel variants with CidB w Pip(Pel) in yeast did strongly enhance levels of the latter protein but only if they were able to bind to it. (Supplementary Fig. 10 )) Thus, these specific residues at the binding interface are particularly important in determining the binding specificity of CidA w Mel . Crystal structure of CidA w Mel (ST)-CidB w Pip(Pel) ND1-ND2 explains interaction specificity We next determined the crystal structure of the CidA w Mel (ST)-CidB w Pip(Pel) ND1-ND2 complex (Supplementary Table 1 and Fig. 3g ). The structure of the complex was very similar to that of CidA w Pip(Tunis) -CidB w Pip(Tunis) ND1-ND2 (RMSD: 0.8 Å over 691 Cα atoms). This structure revealed the interacting residues at the CidA w Mel (ST)-CidB w Pip(Pel) ND1-ND2 interface (Supplementary Fig. 11 ; electron density for representative residues shown in Supplementary Fig. 7 ) and explained why certain CidA w Mel (ST) variants show reduced binding to CidB w Pip(Pel) ND1-ND2 . For example, at region 4, residues R114 and K121 of CidA w Mel (ST) interact electrostatically with residues E460 and D459 of CidB w Pip(Pel) ND1-ND2 , respectively (Fig. 3h ). In CidA w Mel (ST-4), residues 114 and 121 were reverted back to the corresponding residues of CidA w Mel , which are both glutamines (Fig. 3c ). These residues are not charged and may lead to the reduced binding of CidA w Mel (ST-4) to CidB w Pip(Pel) ND1-ND2 (Fig. 3d ). Similarly, at region 7, residues R288 and D299 of CidA w Mel (ST) have charge complementarity with D246 and R252 of CidB w Pip(Pel) ND1-ND2 , respectively (Fig. 3i ). In the CidA w Mel (ST-7) revertant, residues 288 and 299 are glutamine and asparagine, respectively (Fig. 3c ), which can no longer form salt bridges with D246 and R252 of CidB w Pip(Pel) ND1-ND2 . Finally, at region 9, residue R393 of CidA w Mel (ST) interacts with residues E257 and D261 of CidB w Pip(Pel) ND1-ND2 through salt bridges (Fig. 3i ). In CidA w Mel (ST-9), residue 393 is glutamic acid (Fig. 3c ), which cannot bind to E257 and D261 of CidB w Pip(Pel) ND1-ND2 due to electrostatic repulsion. The crystal structure clearly explains the reduced binding of CidA w Mel (ST-4), CidA w Mel (ST-7) and CidA w Mel (ST-9) to CidB w Pip(Pel) ND1-ND2 (Fig. 3d ), which closely parallels their loss of function in yeast growth rescue assays (Fig. 3e, f ). Natural sequence variations affect CidA w Pip(Tunis) -CidB w Pip(Tunis) binding The w Pip cidA-cidB operon is duplicated and diversified extensively among CI-inducing w Pip strains. Interestingly, however, only residues at certain positions are different among the CidA w Pip and CidB w Pip variants [32] (Fig. 4a, b ). If the varied residues are at the CidA w Pip -CidB w Pip binding interface, they may affect the interaction of these proteins and play a role in CI induction and/or rescue specificity. The w Pip Tunis line belongs to group I of w Pip ( w PipI, grouping of w Pip strains is based on phylogenetic analysis of seven Wolbachia genes) [32] , [44] , so we focused on the CidA w Pip and CidB w Pip variants from this group (hereafter, CidA w Pip _I and CidB w Pip _I). (As mentioned before, CidA w Pip(Tunis) and CidB w Pip(Tunis) are CidA w Pip _I(γ/2) and CidB w Pip _I(b/2), respectively.) Fig. 4: Sequence variations modulate interactions between natural CidA w Pip and CidB w Pip alleles. a Sequence alignment shows that residues at certain positions are different among the CidA w Pip and CidB w Pip variants. The residues that are the same among the variants are not shown. The varied residues which are located at the binding interfaces are boxed. The numbers above sequence alignment were based on the sequences of CidA and CidB from w Pip Tunis. b The locations of the varied residues are shown as spheres on the structure of the CidA w Pip(Tunis) -CidB w Pip(Tunis) ND1-ND2 complex. c The varied residues which are located at the binding interfaces are colored and labeled. Other residues at the binding interfaces are shown in gray. d , e His-tagged CidA variants were used to pull down GST-tagged CidB variants. The proteins were detected by Coomassie Blue staining. These experiments were repeated three times independently with similar results obtained. One representative is shown. ND nuclease domain. Source data for panels ( d ) and ( e ) are provided as a Source Data file. Full size image Among the positions that show divergence (Fig. 4b ), residues 118, 125, 149, 150, 341, 342, 399, and 400 of CidA w Pip and residues 242, 243, 253, 254, 257, 451, 452, 460, 461, and 462 of CidB w Pip map to the binding interface of the two proteins (Fig. 4c ). These variations create distinct interaction surfaces for each of the four known CidA w Pip _I variants (Fig. 4a ). Specifically, CidA w Pip variants I(α/1) and I(β/2) have the same residues A118, G125, G149 and G150; the corresponding residues in variants I(γ/1) and I(γ/2) are R118, K125, D149, and S150 (Fig. 4a ). CidA w Pip variants I(α/1) and I(γ/1) both share residues G342, R343, K400, and N401, which correspond to residues Y341, T342, R399, and D400 in variants I(β/2) and I(γ/2). Similarly, each of the four CidB w Pip _I variants has a unique combination of residues at the CidA-binding interface (Fig. 4a ). Pulldown experiments were used to investigate the interactions between the CidA w Pip variants and the CidB w Pip variants. His-tagged CidA variants I(α/1), I(γ/1), I(β/2), and I(γ/2) cannot pull down GST-tagged CidB variants I(b/2), I(b/1), I(a/2), and I(a/1), respectively (Figs. 4d , e ), which supports the hypothesis that natural sequence variations affect binding interactions between CidA w Pip and CidB w Pip from different strains. If binding is required for CidA to rescue CidB-induced defects, this sequence diversity may at least partially explain the complex bidirectional incompatibility patterns in crosses between different C. pipiens lines (discussed below). Here, we have presented structural, biochemical and functional studies on the Wolbachia CI factors CidA w Mel and CidB w Mel , providing a solid foundation for investigation of the molecular functions of the Cid proteins in CI. These proteins are used here as a model to investigate the evolution of CidA-CidB interactions and their biological impact. Our structure-based mutagenesis has led to a clear demonstration of noncognate CifA-CifB binding, which suggests how sequence changes specifically at the interfaces between these proteins could lead to the complex incompatibility relationships that can be observed in the wild [32] . The Cid systems from Wolbachia strains w Mel and w Pip are evolutionarily related, but these strains reside in different clades or supergroups (supergroups A and B, respectively). The two strains are expected to be incompatible based on crosses with trans-infected Ae. albopictus mosquitoes [36] . Here, we show that the CidA-CidB pairs from these Wolbachia strains share the same interaction mode but have different residues at their binding interfaces. These residues are critical for determining their binding specificity. CidA w Mel (ST), a rationally designed chimeric construct containing the scaffold of CidA w Mel and the interfacial residues of CidA w Pip , binds CidB w Pip(Pel) and rescues CidB w Pip(Pel) -induced growth defects in yeast. It proves that CidA variants from different Wolbachia strains use the same pathway to carry out their function. To further evaluate the conservation and evolutionary relationship of CidA and CidB found in different Wolbachia strains, the conservation scores of CidA and CidB residues were calculated by the ConSurf server and mapped onto their structures [45] , [46] , [47] . The residues in the core of the proteins tend to be highly conserved. In contrast, the residues located at the surface are more variable (Supplementary Fig. 4a-b ). Many of the varied residues are located at the CidA-CidB binding interfaces (Supplementary Fig. 4c ). (Although several key residues of CidA at interface III are identical among its homologs, their interaction with CidB cannot be maintained due to residue variations at interface III of CidB.) This agrees with previous hypotheses that the CidA and CidB interfaces are co-evolving [32] , [35] , which could modulate binding between CidA and CidB proteins and lead to incompatibility. Wolbachia strains infecting C. pipiens usually contain more than one copy of the cidA and cidB genes [32] , which has been proposed to be responsible for the very complex incompatible patterns documented in C. pipiens infected with these strains. We showed here that the natural sequence variations in CidA w Pip and CidB w Pip proteins affects their binding specificity. The expression of multiple CidA w Pip and CidB w Pip variants in one Wolbachia strain could lead to a mix-and-match type of binding and may be one reason for the very complex crossing results. The presence of cidB_ IV(2) variants was associated with the incompatible phenotype of mosquitoes infected with group IV w Pip when crossing with those infected with w Pip from other groups [32] , [37] . Indeed, the CidB _ IV(2) variants have unique residues at interface I (including residues 451, 452, 460, 461 and 462) compared to the CidB of the other groups. These differences may impair the binding of the CidB _ IV(2) variants to the CidA variants of the other groups and lead to incompatibility. The crystal structure of CidB w Mel DUB provides a solid structural basis for further investigation of the molecular targets and function of CidB deubiquitylase family proteins. Given that bacteria do not possess a ubiquitin-conjugation system, the presence of a DUB domain in CidB strongly suggests that this Wolbachia protein functions within the host [21] , [40] . Indeed, CidB proteins have been proposed to target nuclear-protein import and protamine-histone exchange factors [48] . CidB w Mel DUB has three variable regions and a C-terminal region different from other bacterial proteases in the CE-clan/Ulp1-like protease family, which could be responsible for its substrate preference for ubiquitin over other ubiquitin-like molecules and for Lys63-linked ubiquitin chains [21] , [40] , [41] . In different models that try to account for how Cif proteins induce and rescue CI, CifA-CifB interaction is suggested to play different roles. In one, which is named the “2-by-1” model, CifB is suggested to have an ancillary role by modulating CifA stability or activity in the male germline [25] . By contrast, in the “toxin-antidote” model, specific CifA-CifB interaction in the egg has been proposed to be essential for CifA to rescue CifB-induced CI [32] , [35] . Two major differences between these models are where CifA and CifB interact (in male or female) and whether the interaction is involved in CI induction or rescue. Our structures of CidA-CidB complexes and attempts to modulate their binding specificity provide a way to rationally design CifA and CifB mutants with desired binding attributes. Analysis of these variants will help distinguish between these and other CI models. DNA manipulation The genes coding for CidA, the variants of CidA, and CidB of w Pip(Tunis), w Pip(Pel) and w Mel were synthesized at the Beijing Genomics Institute (BGI China). These sequences were codon-optimized for expression in E. coli by BGI. For crystallization, CidA w Pip(Tunis) , CidB w Pip(Tunis) ND1-ND2 (residues 1-761), CidB w Pip(Pel) ND1-ND2 (residues 1-761) and CidA w Mel genes were subcloned into the pET-22b(+) vector using restriction sites Nde I and Xho I, encoding proteins with a C-terminal His-tag. CidB w Mel DUB (residues 797-1128) gene was subcloned into the pGEX-6p-1 vector possessing an N-terminal glutathione-S-transferase (GST) tag using restriction sites Bam HI and Xho I. For in vitro pull-down experiments, CidA variants were the same as those used for crystallization. A pET28a-GST vector was made where the GST coding sequence was inserted between restriction sites Nco I and Bam HI on pET28a. The CidB w Pip(Tunis) ND1-ND2 and CidB w Pip(Pel) ND1-ND2 genes were cloned into the pET28a-GST expression vector between restriction sites Eco RI and Xho I so that the proteins expressed had an N-terminal GST-tag. For yeast growth analysis, DNA fragments were subcloned from E. coli vectors by restriction digest or PCR amplification and ligated into yeast expression vectors. The 2-micron plasmid pRS425GAL1 (LEU2) utilizing a GAL1 promoter was used for galactose-induced CifA expression in yeast and the low-copy vector pRS416GAL1 (URA3) was used for galactose-induced CifB expression. 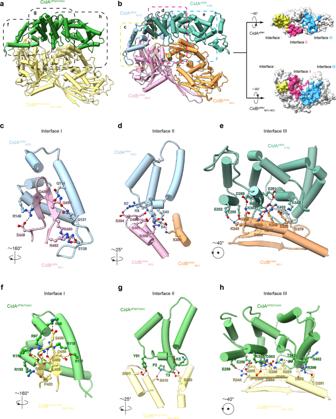Fig. 2: CidA and CidB interact through a large conserved tripartite interface. aThe structure of the CidAwPip(Tunis)-CidBwPip(Tunis)ND1-ND2complex. CidAwPip(Tunis)binds CidBwPip(Tunis)ND1-ND2through three regions (Interface I, II, and III).bA structural model of CidAwMelin complex with CidBwMelND1-ND2was generated by AlphaFold-Multimer. The tripartite interface between CidAwMeland CidBwMelND1-ND2is shown in yellow, magenta and cyan for Interface I, II, and III, respectively.c–eEach interface of the CidAwMel-CidBwMelND1-ND2complex involves a pair of structural motifs. Representative residues directly involving in the interaction are labeled and shown as balls and sticks.f–hThe structural motifs at Interface I, II and III of the CidAwPip(Tunis)-CidBwPip(Tunis)ND1-ND2complex are shown, with residues directly involving in the interaction labeled. NTD N-terminal domain; CTD C-terminal domain; ND nuclease domain. Primers used to generate CifA or CifB expression plasmids are summarized in Supplementary Table 2 . All plasmids were verified by sequencing (Sangon Biotech, China). Protein expression and purification All proteins were expressed in E. coli (BL21 (DE3) strain). Briefly, E. coli transformed with an expressing plasmid was cultured in Luria broth (LB) at 37 °C to an optical density (OD 600 ) of 0.6. Overexpression of the recombinant proteins was induced by adding isopropyl-β-D-thiogalactopyranoside (IPTG) to a final concentration of 0.5 mM at 16 °C for 16–18 h. The harvested bacteria overexpressing CidA w Mel (or CidA variants) were resuspended in a lysis buffer (20 mM Tris-HCl, pH 8.0, 300 mM NaCl, 10 mM imidazole, 10% glycerol) and lysed via a high-pressure homogenizer at 4 °C. The lysate was centrifugated at 26500 × g for 30 min at 4 °C. After centrifugation, the supernatant was loaded onto a Ni-NTA column (GE Healthcare, USA). The column was washed using a lysis buffer supplemented with 50 mM imidazole and eluted using a lysis buffer supplemented with 500 mM imidazole. The eluted protein was diluted with buffer A (20 mM Tris-HCl, pH 8.0, 5 mM DTT) and further purified by anion-exchange chromatography (Hi Trap Q HP 5 mL, GE Healthcare, USA), using a linear gradient of 0%-40% mixture of buffer A and buffer B (20 mM Tris-HCl, pH 8.0, 1 M NaCl, pH 8.0, 5 mM DTT). Finally, the protein was purified by gel-filtration chromatography (Superdex 200 10/300 GL, GE Healthcare, USA), using a buffer containing 20 mM Tris-HCl, pH 8.0, 150 mM NaCl, 5 mM DTT. To obtain the CidA w Pip(Tunis) -CidB w Pip(Tunis) ND1-ND2 and CidA w Mel (ST)-CidB w Pip(Pel) ND1-ND2 complexes, bacterial cells expressing each component of the specific complex were mixed and co-lysed in the lysis buffer containing 20 mM Tris-HCl, pH 8.0, 0.3 M NaCl, 10 mM imidazole, 10 μg/mL DNase 1, 10 μg/mL RNase A and 10% glycerol. The complex were further purified by running cleared lysate sequentially through Ni-NTA affinity, anion-exchange and size exclusion chromatography using the same columns and buffers as described for CidA w Mel . The CidB w Mel DUB protein was purified following a similar procedure, using affinity, anion-exchange and size exclusion chromatography. CidB w Mel DUB has a GST-tag. Instead of using Ni-NTA affinity chromatography, GST affinity chromatography was used. The harvested bacteria overexpressing CidB w Mel DUB were resuspended in a lysis buffer (20 mM Tris-HCl, pH 8.0, 150 mM NaCl, 5% glycerol) and lysed via a high-pressure homogenizer at 4 °C. The lysate was centrifugated at 26500 × g for 30 min at 4 °C. After centrifugation, the supernatant was loaded onto a glutathione-Sepharose column (GE Healthcare, USA). The GST tag was removed by incubating the loaded column with PreScission protease overnight at 4 °C. The CidB w Mel DUB protein was further purified through anion-exchange and size exclusion chromatography using the same columns and buffers as described above. Selenomethionine (SeMet)-derivatized proteins were expressed by bacteria growing in M9 SeMet medium supplemented with 100 mg/L L-selenomethionine. The purification procedure of SetMet-derivated proteins was the same as mentioned above for the native. Crystallization, data collection, and structure determination All crystals were grown by the microbatch-under-oil method unless otherwise specified [49] . CidA w Mel was crystallized at 16 °C by mixing 1 µL protein (5 mg/mL) with 1 µL crystallization buffer containing 0.2 M Sodium phosphate monobasic monohydrate, 20% w/v Polyethylene glycol 3350, pH 4.7. The crystals were cryoprotected by Parabar 10312 (previously known as Paratone oil, Hampton Research, USA). X-ray diffraction data were collected on beamline BL18U1 at the Shanghai Synchrotron Radiation Facility at 100 K and at a wavelength of 0.97852 Å. Data integration and scaling were performed using HKL3000 [50] . The structure was determined by SeMet single-wavelength anomalous dispersion (SAD) method with the AutoSol program in PHENIX [51] . The CidA w Mel model was initially built by the Autobuild program in PHENIX and subsequently subjected to iterative cycles of manual building in Coot [52] and refinement in PHENIX. The crystals of the CidA w Pip(Tunis) -CidB w Pip(Tunis) ND1-ND2 complex were grown at 16 °C from a mixture of 1 µL protein (5 mg/mL) and 1 µL crystallization buffer containing 0.1 M BICINE, pH 8.5 and 15% w/v Polyethylene glycol 1500. The crystals were cryoprotected by Parabar 10312. X-ray diffraction data were collected on beamline BL18U1 at the Shanghai Synchrotron Radiation Facility. The structure was determined by molecular replacement using the structure of the CidA w Pip(Pel) -CidB w Pip(Pel) ND1-ND2 complex as the search model [53] . The crystals of the CidA w Mel (ST)-CidB w Pip(Pel) ND1-ND2 complex were grown at 16 °C from a mixture of 1 µL protein (5 mg/mL) and 1 µL crystallization buffer containing 5% v/v (+/-)-2-Methyl-2,4-pentanediol, 0.1 M HEPES pH 7.5, 10% w/v Polyethylene glycol 10,000. The crystals were cryoprotected by Parabar 10312. X-ray diffraction data were collected on beamline BL18U1 at the Shanghai Synchrotron Radiation Facility. The structure was determined by molecular replacement using the structure of the CidA w Pip(Tunis) -CidB w Pip(Tunis) ND1-ND2 complex as the search model. CidB w Mel DUB was crystallized by hanging drop method at 18 °C, with the crystallization reservoir solution containing 10 mM Nickel (II) Chloride hexahydrate, 100 mM TRIS pH 8.5 and 20% w/v Polyethylene Glycol Monomethyl Ether 2000. The crystals were directly flash frozen in liquid nitrogen using reservoir solution supplemented with 10% glycerol as cryoprotectant. X-ray diffraction data were collected at beamline BL17U1 at the Shanghai Synchrotron Radiation Facility. The structure was determined by SeMet SAD method as described above. Data collection and structure refinement statistics are summarized in Supplementary Table 1 . All Molecular graphics were created using UCSF ChimeraX [54] . In vitro pull-down experiments E. coli BL21(DE3) expressing either His-tagged CidA mutants or GST-tagged CidB ND1-ND2 variants were harvested by centrifugation and resuspended separately in a buffer containing 20 mM Tris-HCl, pH 8.0, 300 mM NaCl, 1 mM PMSF and 5% glycerol. The expression levels of CidA variants were approximated by the BCA Protein Assay (Tiangen Biotech (Beijing) Co., Ltd., China). Equal amount of CidA variants were mixed with a large and fixed volume of CidB ND1-ND2 variants to ensure that CidB ND1-ND2 variants were in excess to CidA. The mixture was co-lysed by sonication. Cleared lysates were incubated with 50 μL Ni-NTA resin at 4 °C for 1 h. The resin was washed eight times with 800 μL buffer containing 20 mM Tris-HCl pH 8.0, 200 mM NaCl, 0.01% Tween-20, 50 mM imidazole each time. Proteins were eluted by adding 3 resin volumes of 20 mM Tris-HCl pH 8.0, 200 mM NaCl, 300 mM imidazole. The samples were analyzed using the SDS-PAGE and Coomassie stain. Yeast growth assays Growth was analyzed in the BY4741 strain as previously described [55] . Briefly, yeast cultures were grown overnight at 30 °C in Yeast Extract Peptone Dextrose (YPD) media or synthetically defined (SD) raffinose media lacking uracil, leucine or both. Yeast were pelleted by centrifugation, washed with sterile water, and spotted in six-fold serial dilution from an initial OD 600 0.2 concentration on solid minimal synthetic media containing either 2% galactose or glucose and lacking either uracil, leucine, or both. Plates were placed at 30 or 36 °C for 2 to 3 days. Western blot analysis For immunoblotting, co-expression culture in raffinose minimal medium (SD) lacking uracil and leucine were diluted to 0.2 OD 600 in galactose (inducing) minimal medium (SD) lacking uracil and leucine, kept 12–16 h at 30 °C until reaching 0.8-1.0 OD 600 at which point the equivalent of 2.5 OD 600 units of cells were harvested, washed and resuspended in 1 mL dH 2 O followed by the addition of 200 μL dH 2 O and 200 μL 0.2 M NaOH, incubated for 5 min at room temperature. Cells were vortexed intermittently for 20 s and pelleted at 10,000 x g, 1 min. Pellets were stored at −80 °C for at least 15 min, resuspended in 100 μL 1 x SDS-PAGE sample buffer and 4% β-mercaptoethanol then heated at 95 °C for 3 min, centrifuged and 20 μL supernatant were loaded in the 10% SDS-PAGE gel and transferred to PVDF Immobilon-P transfer membranes (0.45 μM pore size) (Sigma-Aldrich) under 70 V, 2.5 h used for immunoblot analyses. Antibodies used for immunoblotting were as following: mouse anti-FLAG M2 (Sigma, 1:10,000), secondary antibody used was sheep anti-mouse NXA931V (GE Healthcare, 1:5,000); and mouse anti-PGK1 (yeast phosphoglycerate kinase; Abcam, 1:10,000), secondary antibody used was sheep anti-mouse NXA931V (GE Healthcare, 1:10,000). All immunoblot analyses used 5% milk for blocking. All serial dilution and Western blot data are representative of at least two biological experiments. Proteins were visualized by HRP-based chemiluminescence [56] . AlphaFold modeling In this study, AlphaFold was used to predict the monomer structure of CidB w Mel ND1-ND2 , and AlphaFold-Multimer was used to predict the binding complex of CidA w Mel -CidB w Mel ND1-ND2 with multiple sequence alignments (MSA) set as the all genetics database used at CASP14. The prediction of complexes was run twice with different random seeds and 10 models were obtained. Beginning with visual inspection, four of them were selected to perform protein structural quality check for the side chain conformations using prime module of Schrödinger2021-3. Eventually, the one complex with the highest quality score was selected for further optimization with subsequent MD simulations. Molecular dynamics (MD) simulations MD simulations were performed by using Desmond package of Schrödinger2021-3 [57] using the OPLS4 [58] force field. The binding model of CidA w Mel -CidB w Mel ND1-ND2 obtained in the last step was explicitly solvated with TIP3P [59] water molecules under cubic periodic boundary conditions for a 15 Å buffer region. The overlapping water molecules are deleted and 0.15 M KCl is added, and the systems were neutralized by adding K + as counter ions. Brownian motion simulation was used to relax these systems into local energy minimum states separately. An ensemble (NPT) was then applied to maintain the constant temperature (300 K) and pressure (1.01325 bar) of the systems, and the simulations were started with different random initial velocities. The results were visually analyzed by using Maestro graphical interfaces and the RMSD was calculated based on C-alpha atoms. Produced trajectories were clustered using the Desmond trajectory cluster analysis panel. Finally, the most energetically stable binding complex from the largest cluster of conformation in MD trajectory was selected and minimized again with backbone constraints using the prime module of Schrödinger2021-3. 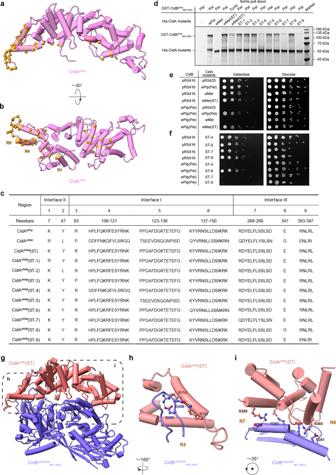Fig. 3: Mutagenesis with binding and yeast growth assays reveal how residues at the three interfaces determine CidA binding specificity. a,bCidAwMel(ST) is a chimera with the body of CidAwMel(pink) and interfacial residues from CidAwPip(Tunis). The locations of the mutated residues are shown in orange on the CidAwMelstructure.cThe substituted residues in CidAwMel(ST) are divided into nine regions (R) and reversed back to those of CidAwMel, individually, to create CidAwMel(ST-1) through CidAwMel(ST-9).dCidAwMel(ST) does not bind wild-type CidBwMelbut binds CidBwPip(Pel)to a similar extent as CidAwPip(Pel). Regions 4, 7, and 9 play important roles in binding. The experiment was repeated three times independently with similar results obtained. One representative is shown.eCidAwMel(ST) is able to rescue yeast from CidBwPip(Pel)-induced lethality.fCidAwMel(ST-4), CidAwMel(ST-7) and CidAwMel(ST-9), which do not bind CidBwPip(Pel), also fail to suppress CidBwPip(Pel)-induced yeast growth defects.gThe crystal structure of the CidAwMel(ST)-CidBwPip(Pel)ND1-ND2complex is similar to the model of the CidAwMel-CidBwMelND1-ND2complex. Representative residues directly involved in the CidAwMel(ST) and CidBwPip(Pel)ND1-ND2interactions at Interface (h) I and (i) III are labeled. ST substituted; ND nuclease domain. Source data for panels (d) and (e) are provided as a Source Data file. 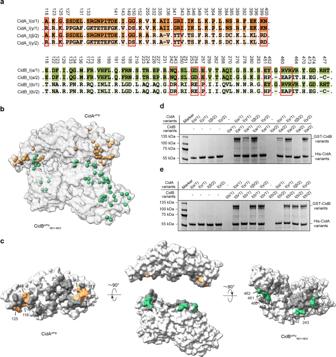Fig. 4: Sequence variations modulate interactions between natural CidAwPipand CidBwPipalleles. aSequence alignment shows that residues at certain positions are different among the CidAwPipand CidBwPipvariants. The residues that are the same among the variants are not shown. The varied residues which are located at the binding interfaces are boxed. The numbers above sequence alignment were based on the sequences of CidA and CidB fromwPip Tunis.bThe locations of the varied residues are shown as spheres on the structure of the CidAwPip(Tunis)-CidBwPip(Tunis)ND1-ND2complex.cThe varied residues which are located at the binding interfaces are colored and labeled. Other residues at the binding interfaces are shown in gray.d,eHis-tagged CidA variants were used to pull down GST-tagged CidB variants. The proteins were detected by Coomassie Blue staining. These experiments were repeated three times independently with similar results obtained. One representative is shown. ND nuclease domain. Source data for panels (d) and (e) are provided as a Source Data file. The Ramachandran plot of the eventual model was generated with Schrödinger2021-3. Evolutionary conservation analysis The conservation score per amino acid of CidA and CidB was calculated using the ConSurf server ( https://consurf.tau.ac.il/ ) based on their homologous sequences (specifically, CidA homologs from WOPip1, WOBol1-b, WOPipJHB, WOHa1, WOSol, WORecB, WOMelB, WOSuziB, and WORiB and CidB homologs from WOPip1, WOBol1-b, WOHa1, WOSol, WOMelB, WOMelPop, and WOSuziB). The structures of CidA w Pip(Tunis) and CidB w Pip(Tunis) ND1-ND2 served as templates. “Maximun likelihood” and “best model” were selected as the calculation method and the evolutionary substitution model, respectively, for this analysis. Reporting summary Further information on research design is available in the Nature Research Reporting Summary linked to this article.